High electron mobility in thin films formed via supersonic impact deposition of nanocrystals synthesized in nonthermal plasmas Thin films comprising semiconductor nanocrystals are emerging for applications in electronic and optoelectronic devices including light emitting diodes and solar cells. Achieving high charge carrier mobility in these films requires the identification and elimination of electronic traps on the nanocrystal surfaces. Herein, we show that in films comprising ZnO nanocrystals, an electron acceptor trap related to the presence of OH on the surface limits the conductivity. ZnO nanocrystal films were synthesized using a nonthermal plasma from diethyl zinc and oxygen and deposited by inertial impaction onto a variety of substrates. Surprisingly, coating the ZnO nanocrystals with a few nanometres of Al 2 O 3 using atomic layer deposition decreased the film resistivity by seven orders of magnitude to values as low as 0.12 Ω cm. Electron mobility as high as 3 cm 2 V −1 s −1 was observed in films comprising annealed ZnO nanocrystals coated with Al 2 O 3 . Controlling charge carrier concentration and mobility in thin films comprising semiconductor nanocrystals is vital for optoelectronic applications. The goal is to achieve the highest possible mobilities with rational control over the majority carrier concentration through doping. While exquisite control over nanocrystal size and size distribution has been achieved in colloidal nanocrystal synthesis, both doping [1] and achieving high mobility in thin films made from these nanocrystals have been challenging. Frequently used synthesis methods for making colloidal nanocrystal leave their surfaces covered with long organic ligands. When thin films are cast from colloidal dispersions of these nanocrystals, the ligands act as insulating barriers and impede charge transport. The nanocrystals can be brought closer together to improve the charge carrier mobilities, either by removing the long-chain ligands or by exchanging them for shorter ones [2] . The presence of electronic surface traps, particularly prevalent in films without surface ligands, also reduces charge mobility. Gating and moving the Fermi level above the trap levels, in films comprising n-type nanocrystals, can fill these traps and increase the charge mobility significantly (as high as 27 cm 2 V −1 s −1 ; refs 3 , 4 , 5 , 6 ). However, gating cannot be used in some important applications such as thin film solar cells and transparent conducting films. Recently, infiltration of the space between the nanocrystals with a coating using atomic layer deposition (ALD) has been shown to be an effective approach for improving the electronic properties of colloidal nanocrystal films. For example, Pourett et al . [7] improved the charge mobility in photodetectors made from colloidal CdSe quantum dot films to 0.01–0.1 cm 2 V −1 s −1 by infiltrating the pores with ALD ZnO, while Liu et al . [8] achieved 6–8 cm 2 V −1 s −1 field effect mobilities in transistors made from PbSe nanocrystals infiltrated with ALD Al 2 O 3 . It is important to note that in all these studies, the effect of traps was eliminated by gating, and the reported mobilities are measured in field effect transistors. In the following, we describe a method for making high mobility (≈3 cm 2 V −1 s −1 ) thin films comprising ZnO nanocrystals synthesized in the gas phase using a nonthermal plasma without ever exposing them to a solvent or surface passivating ligands. While ZnO films comprising nanocrystals have been made [9] , [10] , [11] , [12] , achieving high electron mobility without gating has been elusive. We form thin films comprising these nanocrystals by supersonic expansion and subsequent impaction of the plasma effluent containing the nanocrystals onto suitable substrates. The surfaces of these plasma-synthesized nanocrystals are nominally bare (that is, no ligands) such that the nanocrystals are abutted against each other in thin films formed by supersonic impaction. We show that electronic traps on nanocrystal surfaces can be eliminated in a second process by coating with Al 2 O 3 deposited by ALD. The effectiveness of this strategy is demonstrated in a case study of transparent conducting ZnO. Nanocrystal deposition Zinc oxide nanocrystals were synthesized in the two-stage plasma reactor [13] , [14] illustrated in Supplementary Fig. 1 . The first stage is a nonthermal plasma maintained in a glass tube using radiofrequency electric field: the nanocrystals nucleate and grow in this stage. A slit-shaped nozzle (0.8 × 15 mm) that generates supersonic expansion of the particle-laden gas separates this synthesis stage from the second stage where the substrates to be coated are placed. Experimental details are described in the Methods section. Briefly, ZnO nanocrystals were synthesized from diethyl zinc (DEZ) vapour and oxygen (O 2 ) gas in argon plasma. The DEZ and oxygen were fed in the stoichiometric molar ratio (O 2 :DEZ=7:1) necessary for complete oxidation of DEZ to ZnO, CO 2 and H 2 O. The ZnO nanocrystals synthesized in the plasma were carried to the second stage by the gas flow, which achieves supersonic speeds upon expansion through the slit. The ZnO nanocrystals form a high velocity (100 m s −1 ) particle beam with dimensions slightly larger than the expansion slit and are eventually deposited by inertial impaction onto the substrate immediately downstream of the slit [15] . The substrates were moved back and forth under this beam in a perpendicular direction to the long axis of the slit in a reciprocating motion to simulate a roll-to-roll deposition process. For a given set of flow rates and pressures, the deposition rate depends on the translational velocity and the stroke length; but under typical conditions, the deposition rate was 33 nm s −1 . This is already two to three orders of magnitude higher than the typical deposition rates achieved by sputtering (0.1–1 nm s −1 ) and much higher deposition rates (100–1,000 nm s −1 ) are possible by automation. Deposition rates as high as 200 nm s −1 have shown no ostensible change in the material quality, but the thickness becomes difficult to control reproducibly using manual scanning. Films were deposited on silicon substrates for most characterization experiments but glass substrates were used for electrical and ultraviolet–visible–near infrared (ultraviolet–vis–NIR) transmission measurements. The ZnO nanocrystal films discussed here are 0.4 to 1.0 μm thick. Some films were also annealed at 340 °C in H 2 , which increases the crystallite size (vide infra). Some of the as-deposited and annealed films were also coated with Al 2 O 3 or Al-doped ZnO using ALD. Remarkable differences in the electrical properties of these films are discussed below. Films comprising uncoated nanocrystals The as-deposited thin films comprise densely packed wurtzite ZnO nanocrystals (25–42% packing density). The packing density and the film thickness were determined using spectroscopic ellipsometry. The film thickness and film density were independently checked using scanning electron microscopy (SEM) and Rutherford backscattering. The agreement between the measurements was excellent ( Supplementary Note 1 ) so that fast ellipsometry measurements were used routinely for most samples. The average nanocrystal size, which was tuned in the range from 5 to 7 nm using the residence time in the plasma, was determined from the width of the X-ray diffraction (XRD) peaks using the Scherrer equation ( Fig. 1 , Supplementary Fig. 2 ). 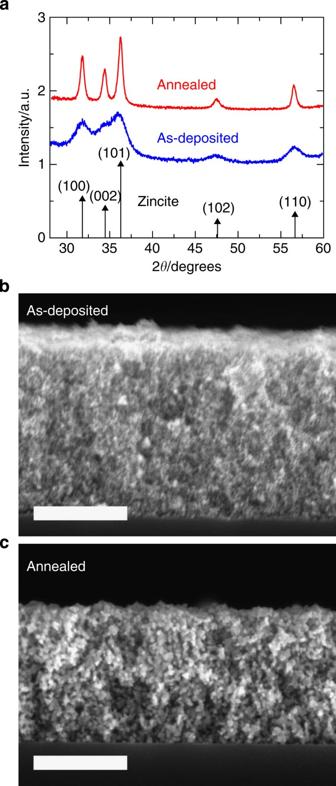Figure 1: Structural characterization of films comprised of uncoated nanocrystals. (a) XRD patterns of ZnO nanocrystals produced using the same plasma synthesis conditions but with different post processing: as-deposited (blue) and after annealing at 340 °C in 20% H2in Ar for 60 min (red). The calculated crystallite sizes (xs) were 4.8±1 nm and 22±5 nm for the as-deposited and the annealed nanocrystal films, respectively. The XRD patterns inahave been offset for clarity. Representative cross-sectional SEM images of ZnO nanocrystal films on silicon substrates processed at the same conditions as panela, (b) as-deposited and (c) after annealing. The scale bars inbandcare 500 nm. Figure 1 shows cross-sectional scanning electron micrographs (SEMs) of an As-deposited and an annealed nanocrystal film deposited under identical conditions. The packing density of this particular As-deposited ZnO nanocrystal film was 25%. After annealing in 20% H 2 in Ar at 340 °C for 60 min at atmospheric pressure, the packing density in the film increased slightly to 31% while the crystallite size increased significantly from 5 to 22 nm. Evidence of this size increase can be seen in Fig. 1 . The electrical resistivities of as-deposited films were very high, >10 9 Ω cm and near the upper limit of our current–voltage measurement system. After annealing in H 2 , the resistivity decreased by three orders of magnitude to 2.9 × 10 6 Ω cm. Figure 1: Structural characterization of films comprised of uncoated nanocrystals. ( a ) XRD patterns of ZnO nanocrystals produced using the same plasma synthesis conditions but with different post processing: as-deposited (blue) and after annealing at 340 °C in 20% H 2 in Ar for 60 min (red). The calculated crystallite sizes ( x s ) were 4.8±1 nm and 22±5 nm for the as-deposited and the annealed nanocrystal films, respectively. The XRD patterns in a have been offset for clarity. Representative cross-sectional SEM images of ZnO nanocrystal films on silicon substrates processed at the same conditions as panel a , ( b ) as-deposited and ( c ) after annealing. The scale bars in b and c are 500 nm. Full size image We discovered that the resistivity of the films improved remarkably when they were placed under vacuum. 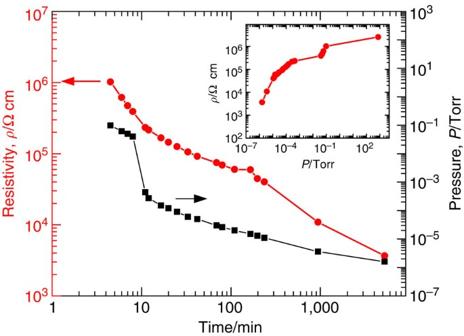Figure 2: Resistivity of an annealed nanocrystal film. Resistivity of an annealed nanocrystal film, prepared using the same conditions as inFig. 1c, as a function of time in a vacuum chamber during pump down (red). The pressure in the chamber as a function of time is the black points. The two curves were combined to give the inset, resistivity as a function of residual air pressure in the vacuum chamber. Figure 2 shows the film resistivity as a function of pressure in a vacuum chamber pumped by a turbomolecular pump (10 −6 Torr base pressure). The resistivity decreased by three orders of magnitude from 3 × 10 6 Ω cm at atmospheric pressure to 4 × 10 3 Ω cm at 1.6 × 10 −6 Torr. Upon venting the chamber, the resistivity returned to its initial value ( Supplementary Fig. 3 ), suggesting that adsorption of a species in air on the ZnO nanocrystal surfaces affects the film resistivity. We hypothesize that an acceptor defect originating from air was reversibly adsorbing to the surface and increasing the resistivity of the ZnO nanocrystal films by trapping electrons and reducing the carrier density. Close examination of Fig. 2 suggests that the ZnO nanocrystal surface coverage of the acceptor remained high and the surface remained approximately saturated until the pressure began to drop below ~0.1 Torr. The steep slope of the data in Fig. 2 at 10 −6 Torr suggests that if the pressure were lowered even further, the resistivity would have continued to drop. Clearly, the cause for the high resistivity of the ZnO nanocrystal films, when measured under ambient conditions, is an adsorbate originating from air whose identity and chemical origin will be proposed shortly. Figure 2: Resistivity of an annealed nanocrystal film. Resistivity of an annealed nanocrystal film, prepared using the same conditions as in Fig. 1c , as a function of time in a vacuum chamber during pump down (red). The pressure in the chamber as a function of time is the black points. The two curves were combined to give the inset, resistivity as a function of residual air pressure in the vacuum chamber. Full size image Films comprising nanocrystals coated with Al 2 O 3 by ALD Figure 2 leads to the hypothesis that the defect originating from air must be removed and the nanocrystal film must be sealed to render the ZnO nanocrystal films conductive and stable. We used ALD to accomplish both these goals. First, we determined the ALD film thickness necessary to infiltrate and fill the pores of the film by measuring the solid volume fraction (using spectroscopic ellipsometry) as a function of ALD film thickness. The pores were filled with ZnO deposited by ALD because it has the same optical properties as the ZnO nanocrystals. We found that the ZnO nanocrystal film reached 90% packing density after 7 nm of ZnO was deposited on the nanocrystals by ALD ( Supplementary Fig. 5 ). The remaining 10% volume was not accessible and the packing density saturated at 90%. Therefore 7–8 nm of ALD films (ZnO, Al-doped ZnO or Al 2 O 3 ) were used to coat the ZnO nanocrystals, resulting in dense cross-sections ( Fig. 3 ). The pores visible in the cross section of the as-deposited film have nearly completely disappeared. Occasional voids account for the remaining 10%. 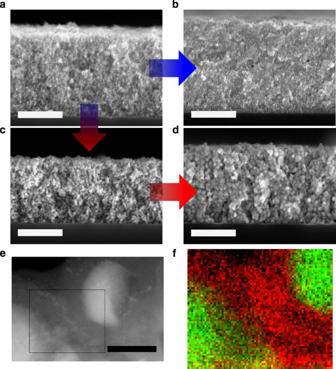Figure 3: Cross-sectional SEM images. Cross-sectional SEM images of as-deposited ZnO nanocrystals on a silicon substrate (a) before and (b) after the nanocrystals have been coated with 7.2 nm of Al2O3using ALD. Annealed ZnO nanocrystals on a silicon substrate before (c) and after (d) coating with 7.7 nm of ALD Al2O3using ALD. (e) Shows a high angle annular dark field scanning transmission electron microscope (STEM) image of annealed ZnO nanocrystals coated with 7.7 nm Al2O3, corresponding tod. (f) Shows a STEM X-ray energy dispersion spectroscopy map of zinc (green) and aluminium (red) distribution in the area defined by the box ine. The scale bars ina–dare 500 nm, andeis 15 nm. Figure 3: Cross-sectional SEM images. Cross-sectional SEM images of as-deposited ZnO nanocrystals on a silicon substrate ( a ) before and ( b ) after the nanocrystals have been coated with 7.2 nm of Al 2 O 3 using ALD. Annealed ZnO nanocrystals on a silicon substrate before ( c ) and after ( d ) coating with 7.7 nm of ALD Al 2 O 3 using ALD. ( e ) Shows a high angle annular dark field scanning transmission electron microscope (STEM) image of annealed ZnO nanocrystals coated with 7.7 nm Al 2 O 3 , corresponding to d . ( f ) Shows a STEM X-ray energy dispersion spectroscopy map of zinc (green) and aluminium (red) distribution in the area defined by the box in e . The scale bars in a – d are 500 nm, and e is 15 nm. Full size image Infilling the ZnO nanocrystal films with 7.7 nm of Al 2 O 3 film deposited through ALD decreased the resistivity by more than seven orders of magnitude. This dramatic decrease upon infilling was observed for both the as-deposited films and the films annealed in 20% H 2 in Ar at 340 °C for 1 h. More specifically, the resistivity decreased by nearly nine orders of magnitude from >10 9 Ω cm to 8.1 Ω cm, while the resistivity of the annealed nanocrystals decreased from 2.9 × 10 6 Ω cm to 0.12 Ω cm. Table 1 summarizes the resistivities of films synthesized using different sequences of post-deposition treatments. Al 2 O 3 is a wide-gap insulator, and it is known that ALD Al 2 O 3 has very high resistivity, ~10 16 Ω cm (ref. 16 ). Thus, we can safely neglect the possibility that any electrical current is flowing through the alumina infill. These low resistivities are achieved without gate bias and measured using direct current in the van der Pauw configuration to eliminate contact resistance ( Supplementary Fig. 7 ). Charge carrier densities and mobilities in the low resistivity films infilled with Al 2 O 3 were determined using Hall-effect measurements. 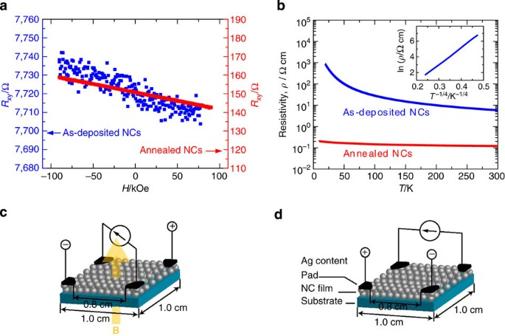Figure 4: Electrical characterization of as-deposited (blue) and annealed (red) films comprised ZnO nanocrystals coated with 7.7 nm of Al2O3using ALD. The average diameters of the as-deposited nanocrystals (blue) and the annealed nanocrystals (red) were 6.5 and 22 nm, respectively. (a) Shows the Hall resistance as a function of magnetic field. The electron concentrations in the as-deposited and the annealed films were 7.6 × 1018cm−3and 1.7 × 1019cm−3, respectively; while the electron mobilities were 0.1 and 3.0 cm2V−1s−1, respectively. Temperature dependence of the resistivity of the films inais shown inb. The inset inbshows that the plot of ln(ρ) versusT−1/4is linear for the as-deposited nanocrystals films, consistent with a Mott 3D VRH electron transport mechanism. (c,d) Show the schematics of the electrode geometry used for Hall effect and van der Pauw sheet resistance measurements, respectively. Figure 4a shows the Hall voltage divided by the source current (that is, the Hall resistance, R xy =V H /I S ) as a function of the magnetic field. The response is linear and shows the classical behaviour expected from an n-type material. The electron mobility in as-deposited ZnO nanocrystal film infilled with Al 2 O 3 was 0.1 cm 2 V −1 s −1 . We caution that such a low value for the mobility means it is probably unreliable. For example, considering the electron effective mass in ZnO is 0.3 m e , a mobility of 0.1 cm 2 V −1 s −1 results in a mean free path of ~4 pm. Considering the radius of Zn 2+ to be 60 pm, such a short mean free path is difficult to interpret physically. More likely the Hall effect has been suppressed because of a hopping electron transport mechanism (see below) for the as-deposited ZnO nanocrystals. When the nanocrystal films are annealed in hydrogen before infilling with Al 2 O 3 , the electron mobility is much higher and increases by a factor of 30 to 3.0 cm 2 V −1 s −1 . This mobility is remarkably high and comparable to electron mobilities in ZnO films deposited by ALD (see below). In fact, the electron mobility is 2% of the values reported for single-crystal ZnO (150 cm 2 V −1 s −1 ; ref. 17 ) and comparable to the electron mobilities in other semiconductor nanocrystal films. For example, Choi et al . [18] measured a field effect electron mobility of 20 cm 2 V −1 s −1 in annealed CdSe nanocrystal films, ~3% of the electron mobility in single-crystal CdSe (660 cm 2 V −1 s −1 ; ref. 17 ). Even without annealing, the electron mobility of the ZnO nanocrystal film, 0.1 cm 2 V −1 s −1 , is 0.07% of the single-crystal mobility; comparable to a recent measurement by Jang et al . [19] , who reported Hall-effect electron mobilities of 16 cm 2 V −1 s −1 in InAs nanocrystal films after rapid thermal annealing, ~0.08% of the electron mobility in single-crystal InAs, 20,000 cm 2 V −1 s −1 (ref. 17 ). Table 1 The properties of films comprising ZnO- and Al 2 O 3 -coated ZnO nanocrystals. Full size table Figure 4: Electrical characterization of as-deposited (blue) and annealed (red) films comprised ZnO nanocrystals coated with 7.7 nm of Al 2 O 3 using ALD. The average diameters of the as-deposited nanocrystals (blue) and the annealed nanocrystals (red) were 6.5 and 22 nm, respectively. ( a ) Shows the Hall resistance as a function of magnetic field. The electron concentrations in the as-deposited and the annealed films were 7.6 × 10 18 cm −3 and 1.7 × 10 19 cm −3 , respectively; while the electron mobilities were 0.1 and 3.0 cm 2 V −1 s −1 , respectively. Temperature dependence of the resistivity of the films in a is shown in b . The inset in b shows that the plot of ln( ρ ) versus T −1/4 is linear for the as-deposited nanocrystals films, consistent with a Mott 3D VRH electron transport mechanism. ( c , d ) Show the schematics of the electrode geometry used for Hall effect and van der Pauw sheet resistance measurements, respectively. Full size image The striking difference between the electron mobility of the annealed nanocrystal network and the as-deposited nanocrystal network (both coated with Al 2 O 3 ) suggests that the transport mechanisms are fundamentally different. To clarify this, we performed temperature-dependent resistivity measurements on both the samples ( Fig. 4b ). The resistivity of the annealed nanocrystal film is nearly independent of temperature and extrapolates to a finite value at 0 K. The value of the resistivity, 0.12 Ω cm, is within a factor of three of an estimate of Mott’s maximum metallic resistivity ( Supplementary Note 2 ). Thus, we conclude that the film is metallic. The critical dopant concentration for Mott’s nonmetal–metal transition in disordered materials is n c =5.7 × 10 18 cm −3 for ZnO ( Supplementary Note 2 ). This is the concentration above which dopants overlap and the material is expected to exhibit metallic conductivity. The electron concentration in the annealed film comprising ZnO nanocrystals coated with Al 2 O 3 is higher than this critical dopant concentration, consistent with the metallic behaviour of the resistivity as a function of temperature. We conclude that the ZnO nanocrystal films are uncompensated, and conduction occurs predominantly by electron transport. In contrast, the as-deposited nanocrystal film shows significant temperature dependence and the resistivity increases with decreasing temperature. The temperature dependence of the resistivity for nondegenerate semiconductors can be described by where T 0 and ρ 0 are constants and the value of m depends on the charge transport mechanism; when m =1, the transport mechanism is band conduction (or in rare cases nearest-neighbour hopping); when m =1/2, the charge transport is either via Efros–Shklovskii variable range hopping or via inter-granular hopping [20] , [21] ; and when m =1/4, the charge transport is via three-dimensional Mott variable range hopping (3D Mott VRH). [22] Using a previously described fitting procedure [20] , we determined that m ≈1/4 for the as-deposited nanocrystal films ( Fig. 4b , Supplementary Fig. 8 ) and, thus, the temperature dependence of the resistivity is consistent with electron transport via the 3D Mott VRH mechanism. We estimated the hopping distance to be 5–10 nm, much smaller than the film thickness, consistent with 3D Mott VRH ( Supplementary Note 3 ). We note that the interpretation of Hall effect data can be complicated in films where the charge transport mechanism is via hopping [20] , requiring caution when comparing various films. While annealing increases the mobility significantly, the electron concentration increases only modestly from 7.6 × 10 18 cm −3 to 1.7 × 10 19 cm −3 suggesting that the lower resistivity in annealed ZnO nanocrystals is primarily due to much higher electron mobility in these films. This increase in mobility is attributed to the significant grain growth that takes place during annealing ( Figs 1 and 3 Supplementary Fig. 2 ). The small increase in electron concentration may be due to a small amount of oxygen vacancies or hydrogen introduced into the film during annealing: both oxygen vacancies and hydrogen could dope ZnO films n-type. Despite the low semiconductor volume fraction and disordered morphology, the annealed and Al 2 O 3 -coated ZnO nanocrystal films exhibit electron mobilities comparable to ZnO films deposited by physical vapour deposition techniques [23] . To shed light on the mechanism by which the ALD Al 2 O 3 is improving the conductivity of the ZnO nanocrystal films, we studied the species present on the nanocrystal surfaces before and after ALD coating, using transmission Fourier-transform infrared (FTIR) absorption spectroscopy. 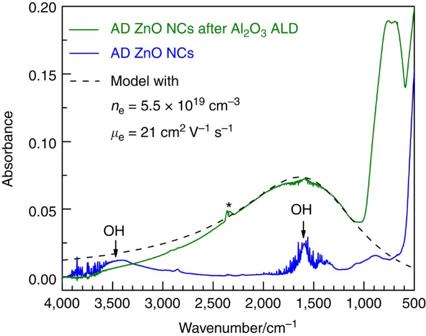Figure 5: FTIR absorption spectra of films comprising as-deposited ZnO nanocrystals on NaCl substrate before (blue) and after (green) coating with 7.7 nm of Al2O3using ALD. The dashed black line is the modelled free carrier absorption of ZnO nanocrystals embedded in Al2O3with electron concentrationne=5.5 × 1019cm−3and mobilityμe=21 cm2V−1s−1. The peak labelled with * is CO2in the spectrometer ambient. The intense absorption between 1,000 and 500 cm−1in the green curve is due to Al2O3. Figure 5 shows the FTIR absorption spectra of a film comprising as-deposited ZnO nanocrystals on a NaCl substrate before and after coating with 7.7 nm Al 2 O 3 . Coating the ZnO nanocrystals with Al 2 O 3 using ALD decreased the surface hydroxide and physically adsorbed water coverage on the ZnO nanocrystals and increased the free carrier absorption. The former appears as absorption peaks at ~3,500 and ~1,600 cm −1 while the latter is a very broad band absorption peaking at ~1,500 cm −1 . It is well known that, in the mechanism for Al 2 O 3 ALD, each ALD cycle is initiated with the reaction of trimethyl aluminium (TMA) with surface hydroxide groups during the exposure of the surface to TMA [24] . TMA reacts readily and irreversibly with the surface OH groups, scavenging them to reduce their coverage significantly. This reduction in the surface OH coverage correlated with the decrease in resistivity of the films deposited on glass ( Fig. 4 and Table 1 ). Moreover, after coating with Al 2 O 3 , the infrared absorption spectrum of the film deposited on the NaCl substrate shows a broad feature consistent with free carrier absorption in ZnO nanocrystals ( Fig. 5 ). Using the Drude–Lorentz–Sommerfield model for the dielectric function and treating the absorption cross-section using Mie theory with the quasi-static approximation for small ZnO particles imbedded in alumina, a theoretical absorption spectrum can be fitted to this broad absorption feature that emerges after Al 2 O 3 coating ( Supplementary Note 4 ). Fitting the theoretical absorbance spectrum to the measured FTIR spectrum yields an electron concentration of 5.5 × 10 19 cm −3 , in reasonable agreement with the Hall measurement, and an electron mobility of 21 cm 2 V −1 s −1 . The higher electron mobility compared with the Hall measurement is expected because optical absorption probes the local conductivity within a ZnO nanocrystal and does not include the reduction in mobility because of grain boundary scattering. The FTIR data shown in Fig. 5 are also consistent with the reversible decrease in resistivity of uncoated ZnO nanocrystal film when it is placed under vacuum ( Fig. 2 ). The width of the depletion layer expected to form after the equilibration of the Fermi level with surface defects is larger than the nanocrystal size, suggesting that the nanocrystals would be completely depleted of electrons in presence of the surface defects ( Supplementary Note 5 ). This is consistent with the high resistivity in films comprising uncoated ZnO nanocrystals. All these experiments support the hypotheses that surface hydroxide groups, originating from reversible water adsorption, are acting as acceptor defects. The elimination of these surface defects is clearly critical to producing conductive ZnO nanocrystal networks. Figure 5: FTIR absorption spectra of films comprising as-deposited ZnO nanocrystals on NaCl substrate before (blue) and after (green) coating with 7.7 nm of Al 2 O 3 using ALD. The dashed black line is the modelled free carrier absorption of ZnO nanocrystals embedded in Al 2 O 3 with electron concentration n e =5.5 × 10 19 cm −3 and mobility μ e =21 cm 2 V −1 s −1 . The peak labelled with * is CO 2 in the spectrometer ambient. The intense absorption between 1,000 and 500 cm −1 in the green curve is due to Al 2 O 3 . Full size image We have considered alternative hypotheses for the remarkable increase in the ZnO nanocrystal film conductivity on annealing and Al 2 O 3 coating. One possibility is that Al from Al 2 O 3 diffuses into and dopes the ZnO nanocrystals. However, the diffusion coefficient for Al in ZnO is ~10 −32 cm 2 s −1 at 180 °C, the ALD temperature [25] . Thus, we eliminate diffusion of and subsequent doping with Al as a possible mechanism that can increase the conductivity. A second possibility is that the Al 2 O 3 film, or the ALD process, injects oxygen vacancies into the ZnO nanocrystals. While the oxygen vacancy diffusion coefficient is larger than that of Al, it is still very small, ~2.4 × 10 −25 cm 2 s −1 at 180 °C (ref. 26 ). Additional evidence against any hypotheses based on the creation and diffusion of a dopant into the ZnO nanocrystal films is that the electron concentration in the annealed ZnO nanocrystal film is higher than that in the as-deposited film even though the annealed nanocrystals are much larger: larger crystals have much smaller surface-area-to-volume ratio and doping by diffusion from the coating is expected to be most effective for films comprising smaller nanocrystals. A third possibility is that the Al 2 O 3 layer results in some type of interfacial doping or a layer of oxygen vacancies that then creates an interfacial electron gas [27] , [28] . We neither have any evidence for such a mechanism nor can completely rule it out. A related hypothesis is that heterogeneous doping [29] , [30] is increasing the electron concentration in the ZnO with Al 2 O 3 coating by inducing oxygen vacancies in the ZnO, but, again, we have do not have direct supporting evidence nor can we completely rule it out. However, these hypotheses appear to be inconsistent with the fact that annealed ZnO nanocrystals coated with Al 2 O 3 have larger electron concentration, despite their lower surface-area-to-volume-ratio, than the as-deposited nanocrystals coated with Al 2 O 3 . Films comprising nanocrystals coated with Al:ZnO by ALD Finally, from a technological perspective, it is interesting to view the two-step process comprising nanocrystal film deposition followed by ALD as a way of increasing the mass deposition rate of ALD processes. As ALD films are ideally conformal everywhere on the nanostructured surface, the mass deposition rate increases with the increased surface area provided by the nanocrystals: the surface area available for ALD divided by the substrate area is very high (~10 2 to 10 3 × ). Consequently, significantly fewer ALD cycles are necessary to deposit a given film thickness [31] . This simultaneously increases the overall deposition rate of the ALD process and reduces the amount of precursor waste, since fewer cycles are necessary and some fraction of the precursor is wasted in each cycle. To demonstrate this idea, 15 nm of Al:ZnO was deposited, using ALD, on the annealed ZnO nanocrystals comprising a 0.38 μm thick film. The Al:ZnO deposited by ALD, like the Al 2 O 3 , infiltrates and fills the void spaces in the nanocrystal film as shown in Supplementary Fig. 10 . The sheet resistance of the Al:ZnO film created using a combination of ZnO nanocrystal deposition followed by 15 nm of Al:ZnO ALD infilling is a factor of 70 lower than the sheet resistance of the 15-nm thick Al:ZnO film deposited directly onto a glass substrate using only ALD (99 Ω per square and 7,000 Ω per square, respectively). It takes 1,000 ALD cycles to reach a sheet resistivity similar to that achieved using a combination of ZnO nanocrystal deposition followed by 15 nm of Al:ZnO ALD, which requires only 100 cycles. The resistivity of ZnO nanocrystal film coated with 15 nm of Al:ZnO is similar to that of the Al:ZnO film deposited directly on glass, but the former was made using a factor of 10 fewer cycles ( Table 2 ). All the Al:ZnO films are more resistive than Sn:In 2 O 3 , but the advantage of ZnO-based materials is that zinc is much less expensive and more abundant than indium. All the films were transparent in the visible region of the spectrum ( Supplementary Figs 9 and 11 ). Table 2 Comparison of the sheet resistance, R s , and resistivity of films comprising ZnO nanocrystals coated with Al:ZnO using ALD (rows 1,2) and Al:ZnO films deposited directly on glass substrates with ALD (rows 3,4). Full size table In conclusion, a nonthermal plasma-based gas-phase approach to depositing thin films comprising ZnO nanocrystals was demonstrated. Nanocrystals synthesized in the plasma are accelerated by supersonic expansion of the plasma effluent and deposited on suitable substrates by impaction without exposure to solvents. Annealing 5 nm ZnO nanocrystals in 20% hydrogen in argon at 340 °C resulted in grain growth to 22 nm and a small decrease in resistivity. Coating the ZnO nanocrystals with 7 to 8 nm of Al 2 O 3 decreases the resistivity by seven orders of magnitude. This decrease is observed both for as-deposited and annealed nanocrystals. Films comprising nanocrystals coated with Al 2 O 3 are n-type with an electron mobility of 0.1 cm 2 V −1 s −1 and 3.0 cm 2 V −1 s −1 for as-deposited and annealed ZnO nanocrystals, respectively. Ultrasensitivity of the resistivity to ambient air and FTIR measurements support the hypothesis that OH on the surface act as an electron trap. Reaction with TMA during ALD of Al 2 O 3 on the ZnO nanocrystals removes these OH traps. Moreover, the Al 2 O 3 coating prevents subsequent adsorption from the ambient. Transparent conducting thin films comprising ZnO nanocrystals coated with Al:ZnO using ALD had similar resistivity and transparency to Al:ZnO films deposited directly on glass using only ALD, but the former required an order of magnitude fewer cycles. Plasma synthesis Supplementary Figure 1 shows the schematic of the two-stage process used to deposit the films comprising ZnO nanocrystals. The two stages are separated by a slit that expands the gases from the first stage into the second stage supersonically. The nanocrystals are synthesized in the nonthermal plasma maintained in a 1′′ glass tube (0.75′′ inner diameter), which comprises the first stage. Diethyl zinc (DEZ, Sigma-Aldrich, Saint Louis, MO), and molecular oxygen (O 2 ) were used as the Zn precursor and the oxygen source, respectively. The flow rates of all the gases were controlled with mass flow controllers (MKS 1179 series and Edwards model 825 series B). The DEZ, a volatile liquid at room temperature, was fed into the plasma using a bubbler and Ar as the carrier gas. The DEZ flow rate was determined from the flow rate of argon into the DEZ bubbler, the DEZ vapour pressure at the bubbler temperature (298 K), the total bubbler pressure (80 Torr) measured using a capacitance manometer (Baratron model 727A, MKS, Andover, MA), the ideal gas law and the law of mass conservation. The DEZ- and O 2 -containing streams were fed into the plasma separately. The DEZ carried by argon was injected through the side port while the oxygen diluted in argon was fed into the plasma through the top port ( Supplementary Fig. 1 ). The flow rates of DEZ, Ar and DEZ, O 2 and Ar, and O 2 were F DEZ =4 s.c.c.m., F Ar,DEZ =20 s.c.c.m., F O2 =30 s.c.c.m., F Ar,O2 =250 s.c.c.m., respectively, where s.c.c.m. is the volumetric flow rate in cm 3 min −1 at 273 K and 1 atm. Mass flow rate can be calculated from the volumetric flow rate at standard conditions and the process conditions using the ideal gas law. The pressure in the plasma ( P 1 , that is, in the first stage) was 3.6 Torr for most of the experiments in the article, but was raised to 5.6 Torr to synthesize the as-deposited ZnO nanocrystals discussed in Figs 4 and 5 as well as in Table 1 ; the increase in pressure was necessary to increase the residence time and, therefore, the crystallite diameter, d p , from d p =5 nm at 3.6 Torr to d p =6.5 nm at 5.6 Torr. The residence time to synthesize the 5 and 6.5 nm nanocrystals were ~27 and 42 ms, respectively. The plasma was generated and maintained by applying a radiofrequency electric field at 13.56 MHz, through a custom impedance matching network, to a copper ring electrode wrapped around the top port ( Supplementary Fig. 1 ) just above the zone where the DEZ-containing and O 2 -containing streams are mixed (hereafter referred to as the mixing zone). The quick disconnect fitting forming the vacuum seal above the deposition stage chamber (that is, the second stage) is the closest grounded surface to the powered electrode and thus served as the ground electrode. The plasma extended ~10 cm downstream of the mixing zone. Approximately 30 cm downstream of the mixing zone was a rectangular slit-shaped orifice with a cross-sectional area of 0.8 × 15 mm. As mentioned earlier, two different orifices were used that had the same cross-sectional dimensions but different lengths in the direction of flow. The orifice for a plasma pressure of 3.6 Torr (5 nm particles) was 2 mm long, and, for a plasma pressure of 5.6 Torr (6.5 nm particles), the orifice was 10 mm long. The deposition stage downstream was a chamber evacuated by a Leybold Turbovac 1000C turbo pump. The pressure in the second stage was P 2 =14 × 10 −3 Torr. Thus, the ratio of the pressure upstream of the slit to the pressure downstream of the slit ( P 1 / P 2 ) was either 257 or 400, depending on the upstream pressure ( P 1 =3.6 Torr or 5.6 Torr, respectively). At these ratios, the flow through the slit was choked and the gas underwent supersonic expansion downstream of the slit where the particle beam forms. In the deposition chamber (that is, the second stage), the substrates were mounted to a push-rod (CRPP-1, MDC vacuum, Hayward, CA) and moved back and forth under the particle beam in a reciprocating motion to simulate a roll-to-roll process. The frequency of the reciprocating motion was ~1 Hz, and the stroke length was ~4 cm. In a typical experiment, films were deposited on two substrates simultaneously, one polished silicon and the other Corning Eagle XG borosilicate glass (MTI Corporation, Richmond, CA). Each substrate was ~1 × 1 cm 2 . The films on glass substrates were used for electrical and ultraviolet–vis–NIR transmission spectroscopy characterization while the films on the silicon substrates were used for XRD, spectroscopic ellipsometry and electron microscopy. The films were deposited on NaCl substrates for characterization with FTIR transmission spectroscopy. Annealing Some films were annealed before ALD in a tube furnace in 500 s.c.c.m. of 20% H 2 and 80% Ar gas flow. During annealing, the substrates coated with the nanocrystal films were placed in a 1′′ outer diameter quartz tube inserted within the tube furnace at room temperature. First, the tube was purged for 30 min at room temperature to remove the air within the tube volume. Then, the power to the heater was turned on and the furnace temperature increased to 340 °C over a period of ~25 min. This temperature was maintained under flowing gas for 60 min. At the end of this period, the power was turned off and the furnace was allowed to cool at the natural cooling rate of the system. The substrates coated with the films were removed once the furnace temperature decreased below 40 °C, which took ~3 h. Atomic layer deposition A commercial reactor (Savannah S200, Cambridge Nanotech/Ultratech, Waltham, MA) was used for ALD. All depositions were conducted at 180 °C. Before precursor pulsing, the films comprising ZnO nanocrystals were allowed to outgas for 2,000 s at 0.5 Torr (also the deposition pressure) in nitrogen gas flowing over the film at 20 s.c.c.m. Nitrogen was also used as the carrier gas during deposition. TMA was used as the aluminium source and DEZ was the zinc source. Each ALD cycle for all depositions in this article consisted of 0.1 s H 2 O pulse followed by 30 s purge and 0.1 s metal–organic precursor (DEZ or TMA) pulse followed by 30 s purge. These steps were repeated periodically to deposit the desired film thickness. For doping ZnO with Al (that is, Al:ZnO deposition), the super-cycle strategy was used [16] , [32] . One super-cycle consisted of 19 cycles of ZnO followed by one cycle of Al 2 O 3 . The 15 nm Al:ZnO film was deposited using five super-cycles, which results in a total of 100 ALD cycles. The substrates with the films were removed from the reactor after coating and allowed to cool in air. Structural characterization The films on silicon were characterized by a variety of techniques. Film thickness and ZnO volume fraction were measured using spectroscopic ellipsometry (J. A. Woollam M44). The Bruggeman effective medium approximation was used to model the optical properties of film and to extract the ZnO volume fraction and film thickness. The film was assumed to be comprised of ZnO and voids. The spectra were fit in the wavelength region between 450 and 750 nm where no size effects on the optical constants of ZnO are expected and the nanocrystal film is transparent. In select experiments, the areal atomic density measured by spectroscopic ellipsometry (that is, film thickness × ZnO volume fraction) was compared with that measured by Rutherford backscattering, and the two measurements were found to be in excellent agreement for ZnO volume fractions greater than ~1% ( Supplementary Fig. 4 ). X-ray diffraction (Cu Kα) from the films was collected using a beryllium area detector in a Bruker D8 Discover diffractometer. The crystallite size was determined from the full-width-at-half maximum of the XRD peaks after subtracting the instrumental broadening, and then using the Scherrer equation. Films were examined using SEM in a JEOL 6700 FEG SEM operating at 5 keV accelerating voltage. The silicon substrates with nanocrystal films were cleaved and mounted on the sample holder such that the substrate surface onto which the nanocrystals were deposited was parallel to the electron beam for cross-sectional imaging. Ultraviolet–vis–NIR spectroscopy was carried out in a Cary 5000 (Agilent Technologies, Santa Clara, CA) in transmission mode using the transmission of a blank glass substrate for the baseline. FTIR spectra were collected in a Nicolet Magna IR 550 (Thermo Scientific, Madison, WI) in transmission mode using an uncoated bare NaCl substrate as the background. The sample compartment was allowed to purge for 2.5 min with dry and CO 2 -scrubbed air before acquiring data. Resistivity measurements The electrical resistivity measurements were carried out in a cryomicroprobe station (Janis Research, Wilmington, MA) with the probes connected to an Agilent 4155C semiconductor parameter analyzer. The probe station was equipped with a turbo pump for pressure-dependent measurements, which was used in select experiments. All reported resistivity values were measured at room temperature and pressure, unless otherwise stated (for example, Figs 2 and 4b ). Silver electrodes, 500 nm in thickness, were deposited on top of the nanocrystal thin films by thermal evaporation at a rate of 2 nm s −1 . For low resistivity samples, the van der Pauw electrode configuration was used to measure the sheet resistance. For high resistivity samples, the electrode configuration was two parallel stripes (1.0 × 0.1 cm) each at the opposite edges of the 1 × 1 cm 2 glass substrate. Temperature-dependent resistivity measurements were done using soldered In contacts to evaporated Ag contact pads in a four-wire van der Pauw configuration. Measurement was made using direct current excitation. The temperature of the sample was controlled using a Janis close-cycle refrigerator. Extensive checks were made at several temperatures during the experiment to ensure ohmic behaviour, account for contact resistance and minimize joule heating. Transmission electron microscopy Electron-transparent specimens (deposited on Si substrate) for cross-section TEM were prepared by the small-angle cleaving technique. This technique relies on thinning a crystallographic substrate to the point that it can be fractured along non-preferred crystallographic plane at a shallow to an easy-cleave plane resulting in a long, thin wedge whose tip is electron transparent [33] . Bulk samples were cleaved to smaller than 1 cm 2 and bonded film-side down to a parallel polishing fixture using CrystalBond 509. The samples were thinned to l<100 μm using an Allied Multiprep and 30 μm diamond lapping film. The sample was oriented in the polishing direction such that scratches were aligned ~10° from the easy-cleave [110] direction. Using a metal ruler and diamond scribe, deep scratches were created along the polishing direction ~1 mm apart. The sample was removed from the polishing fixture using acetone and placed in a petri dish containing a glass slide. Using tweezers, the specimen was carefully cleaved along the scratches using the tweezers and edge of the glass slide. These pieces were then cleaved again along the easy-cleave plane using the tweezers and edge of the glass slide. Samples having a sharp tip were mounted to slot-type Mo TEM grids using MBond 510 epoxy. Cross-section high-angle annular dark field scanning transmission electron microscopy (HAADF-STEM) micrographs and energy dispersive X-ray spectroscopy (EDX) maps were acquired in an aberration-corrected FEI Titan 60-300 (S)TEM equipped with an Analytical SuperTwin pole piece and SuperX EDX detector operating at 300 kV and having a STEM convergence angle of 30 mrad, 150 pA probe current and 58.5 mrad HAADF inner angle. EDX maps were acquired using the Bruker Esprit software with a 612 by 612 pixel frame, 55 μsec pixel dwell time and 23 frames for a total acquisition time of 475 s. EDX net count maps of the Zn Kα and Al Kα peaks were generated using the Esprit software with elemental consideration of zinc, aluminium, oxygen, silicon, carbon and copper. Trace silicon and carbon peaks are a result of the silicon substrate and specimen contamination, respectively, while copper is a result of the TEM grid. Hall measurements Hall measurements on films comprising ZnO nanocrystals coated with Al 2 O 3 were conducted at 300 K in a Quantum Design Physical Properties Measurement System equipped with a 9 T superconducting magnet. Electrical contact to the films was made with In on Ag contact pads evaporated onto the sample in the van der Pauw configuration. Current–voltage characteristics were measured with a Keithley 220 programmable current source and a Keithley 2000 multimeter to measure voltage. In all the cases, extensive checks were made to ensure ohmic behaviour, account for contact resistance and minimize joule heating. Hall measurements on the AZO-coated nanocrystal films were also carried out at 300 K utilizing an electromagnet up to a 0.6 T field. These films were contacted with In contacts, again in the van der Pauw configuration, and current–voltage characteristics were measured using alternating current techniques (16 Hz). How to cite this article: Thimsen, E. et al . High electron mobility in thin films formed via supersonic impact deposition of nanocrystals synthesized in nonthermal plasmas. Nat. Commun. 5:5822 doi: 10.1038/ncomms6822 (2014).